Multimode laser cooling and ultra-high sensitivity force sensing with nanowires Photo-induced forces can be used to manipulate and cool the mechanical motion of oscillators. When the oscillator is used as a force sensor, such as in atomic force microscopy, active feedback is an enticing route to enhance measurement performance. Here we show broadband multimode cooling of −23 dB down to a temperature of 8±1 K in the stationary regime. Through the use of periodic quiescence feedback cooling, we show improved signal-to-noise ratios for the measurement of transient signals. We compare the performance of real feedback to numerical post processing of data and show that both methods produce similar improvements to the signal-to-noise ratio of force measurements. We achieved a room temperature force measurement sensitivity of <2 × 10 −16 N with integration time of less than 0.1 ms. The high precision and fast force microscopy results presented will potentially benefit applications in biosensing, molecular metrology, subsurface imaging and accelerometry. To attain high-resolution mass, position and force sensing, cantilevers with low effective masses and high mechanical quality factors are required. Nanoscale resonators are excellent candidates for mass and force sensing [1] , [2] , [3] , biomaterial sensing by means of Kelvin probe force microscopy [4] and single-spin and charge detection [5] . Miniaturized oscillators, however, are more susceptible to thermal noise and their use can be challenging as it entails low-noise, high-frequency electronics to monitor and control the vibrational modes. Passive cooling is not always an option, particularly in biomaterial sensing applications where samples are dependent on specific environmental conditions. Active feedback cooling can instead be used to reduce the Brownian motion of the oscillators. To date, effective optical cooling of micro/nanomechanical resonators has been achieved via cavity cooling [6] , [7] , [8] and active optical feedback cooling [9] through radiation pressure [10] , [11] , [12] , [13] and photothermal [14] , [15] forces. A feedback system will suppress all motions of the oscillator and has no way to differentiate between motion because of thermal noise and a signal that one wishes to detect. The signal-to-noise ratio (SNR) of the sensor under conditions of steady-state feedback therefore may not be straightforwardly enhanced [16] . Not all is lost, however, as the increased effective damping rate because of feedback can give the oscillator a larger linewidth, which means that the oscillator will respond more quickly to external forces. As a result, less integration time is required to detect steady-state signals with the adoption of feedback cooling [17] . Feedback cooling requires constant measurement of the system in order to generate a control signal to counteract thermalization. If these measurement data are not used for feedback, one may ask whether the data can still be used to improve our knowledge of the system dynamics and the measurement outcome. Provided that we are dealing with linear systems, these measurement data can indeed be fed into numerical estimation algorithms such as Kalman or Wiener filters. These techniques allow tracking and prediction of the motion, which can yield advantages similar to those of feedback cooling. In fact, it is possible to use numerical algorithms to simulate the effect of physical feedback cooling [18] . These estimation techniques require accurate knowledge of the system parameters to perform efficiently. In a nanoscale optomechanical system, the phase and amplitude noise of the laser can alter the system parameters [19] and real-time tracking may be required for optimum estimation. Outside the confines of the steady-state regime, feedback and estimation can be used to improve the SNR [16] , [18] . To date, active cooling of nanomechanical systems in the transient regime has not been observed and its implications for impulsive force sensing have not been studied. In the presence of an impulsive force, feedback cooling can be turned on before measurement and then turned off during the measurement. This periodic quiescence feedback works in such a way that the effect of an impulsive external force on the resonator is measured before the system is fully thermalized. In this case, the SNR of a pulsed signal can be improved by synchronizing the feedback in cycle with the signal. As with the steady-state conditions, it has also been predicted that an equivalent enhancement can be achieved by using estimation techniques, provided the system dynamics are well known (see Supplementary Information of ref. 18 ). In this letter we investigate the dynamics of gold-coated Ag 2 Ga nanowires ( http://nauganeedles.com ). Using homodyne detection we can measure the motion of the nanowire and then actively control the vibration of its modes using bolometric forces. Our set-up is cavity-free, allowing cooling to be accomplished over a wider bandwidth where simultaneous cooling of multiple vibrational modes [20] is observed. We explore the implementation of non-stationary active cooling on nanomechanical oscillators by means of optical forces and observe SNR enhancement of impulsive force measurements. We then compare the results with off-line estimation techniques and show enhancement by a factor of about 5 using periodic feedback cooling as well as estimation methods. Using both physical control and estimation techniques we achieved a force sensitivity of better than 2 × 10 −16 N. Detection and feedback The experimental set-up is presented in Fig. 1a , with scanning electron microscopy images of a nanowire shown in Fig. 1b (for more details on its properties and characterization refer to Supplementary Note 1 ). Optomechanical cooling often relies on optical cavity resonators to enhance the coupling to the mechanical modes. In that case the operational bandwidth is limited by the cavity dynamics and allows only a single mechanical frequency to be addressed via optical interaction. In our experiment, we use a microscope objective to maximize the single-pass interaction of the nanowire with the laser light. The absence of a cavity allows simultaneous access to all of the nanowire’s mechanical resonances. Light scattered from the nanowire is used in a homodyne measurement system [9] . The motion of the nanowire is therefore referenced to the phase of the detection laser. The SNR of this measurement is limited by the amount of scattering from the nanowire. The power used in the measurement is low enough to prevent the observation of any back-action because of the detection laser. 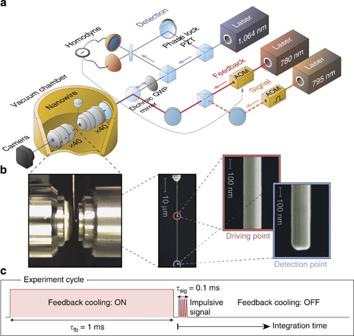Figure 1: Schematic of experimental set-up and experiment cycle. (a) Experimental set-up. The position of the nanowire is controlled by a nanopositioning stage. One laser (1,064 nm) acts as a detection beam. Reflected and transmitted light from the nanowire are detected using a balanced homodyne and camera, respectively. Light is focused on, and collected from, the nanowire using a pair of microscope objectives ( × 40, NA=0.65). A second laser (780 nm) is intensity-modulated using an acousto-optic modulator, enabling feedback actuation based on the homodyne signal. During transient regime measurements, a third laser (795 nm) modulated to provide the impulsive signal is used. (b) Mounting arrangement and scanning electron microscope close-ups of a cylindrical Ag2Ga nanowire ~60-μm long and 150-nm thick. The detection beam interacts with the free end of the nanowire while the feedback or impulsive signal driving beams are typically positioned ~10 μm from the tip to enhance the thermal bending. (c) Schematic of the experiment duty cycle during transient cooling and impulsive force measurement. Figure 1: Schematic of experimental set-up and experiment cycle. ( a ) Experimental set-up. The position of the nanowire is controlled by a nanopositioning stage. One laser (1,064 nm) acts as a detection beam. Reflected and transmitted light from the nanowire are detected using a balanced homodyne and camera, respectively. Light is focused on, and collected from, the nanowire using a pair of microscope objectives ( × 40, NA=0.65). A second laser (780 nm) is intensity-modulated using an acousto-optic modulator, enabling feedback actuation based on the homodyne signal. During transient regime measurements, a third laser (795 nm) modulated to provide the impulsive signal is used. ( b ) Mounting arrangement and scanning electron microscope close-ups of a cylindrical Ag 2 Ga nanowire ~60-μm long and 150-nm thick. The detection beam interacts with the free end of the nanowire while the feedback or impulsive signal driving beams are typically positioned ~10 μm from the tip to enhance the thermal bending. ( c ) Schematic of the experiment duty cycle during transient cooling and impulsive force measurement. Full size image The actuation laser has a different wavelength to the detection laser to avoid any chance of interference between these subsystems. The dominant force on the nanowire is bolometric, that is, it results from differential thermal expansion of a bimorph structure [21] , [22] , [23] . In our case, it is the composite Au/Ag 2 Ga structure of our nanowires that leads to strong thermal effects. The speed of the force depends on the thermal time constant of the object being heated; therefore, it is naturally slow for macroscopic oscillators. For nanoscale objects, however, it can be both fast and substantial in magnitude [24] , [25] . The response time of the nanowire to laser driving is found to be 15 μs at ambient pressure. Unlike radiation pressure, the direction of the force depends only on the structure of the object and is independent of the direction of the incident beam that is used to drive the nanowire. Experimental evidence of these aspects is offered in Supplementary Notes 2 and 3 and Supplementary Figs 1–4 . Bolometrically actuated feedback cooling is somewhat counterintuitive, as the amplitude of the oscillations is subdued by use of a driving force of thermal origins—effectively cooling by heating. Even so, recent theoretical work shows that photothermal effects can assist cooling towards the quantum ground state [26] , [27] , [28] and photothermal back-action in a cavity has also been used to cool a semiconductor membrane [15] and a graphene sheet [14] . 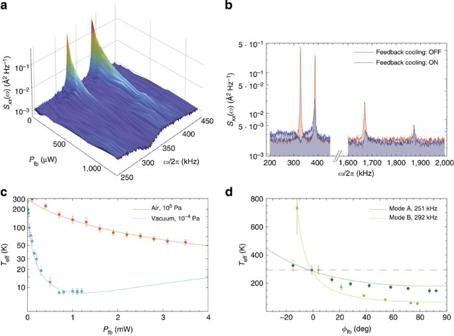Figure 2: Experimental results of multimode photothermal cooling of a nanowire. (a) Displacement spectrum of the two orthogonal fundamental modes of a nanowire (R≈100 nm,L≈40 μm) for different powers of the feedback beam at vacuum condition (10−4Pa). (b) Simultaneous cooling of four distinguished resonances of the nanowire in vacuum with phase and gain optimized for more efficient cooling on one mode per pair. The displacement spectrum data in the absence of feedback is in red and the trace with feedback cooling is in blue. (c) Effective temperature of the first vibrational mode as a function of feedback laser power at ambient (red) and vacuum (blue) conditions. The solid line represents the theory assuming a linear relation between laser power and feedback gaing. (d) Effective temperature of the first (dark-green) and second (light-green) vibrational modes as a function of the phase of the feedback signal. Phases of −90° and 90° correspond to maximum oscillation amplification and maximum cooling, respectively. The solid lines represent the theory predictions. The error bars inc,dare estimated based on error propagation in the Lorentzian fit of the amplitude noise. Figure 2a shows the displacement spectrum of the nanowire for increasing power of the feedback beam under vacuum conditions. The phase of the feedback is adjusted using an adjustable bandpass analogue filter. The feedback phase can be tuned such that simultaneous cooling of multiple modes of the nanowire can be obtained, as seen in Fig. 2b where we plot the uncooled (red) and cooled (blue) vibrational modes of the nanowire up to 2 MHz for a particular phase and gain of the feedback loop. Applying a more advanced RF phase shifter, it is in fact feasible to efficiently cool vibrational modes over a broader frequency range. A comparison of the best effective temperatures reached under ambient and vacuum conditions is plotted as a function of feedback strength in Fig. 2c ; we have achieved cooling greater by an order of magnitude and for reduced driving power in vacuum compared with ambient pressure because of the improved mechanical quality factor. Figure 2d shows the relation between phase and cooling for the first two oscillation modes of a nanowire under ambient pressure conditions; the difference in efficiency is attributed to dissimilarities in geometrical qualities along the directions of oscillation. Figure 2: Experimental results of multimode photothermal cooling of a nanowire. ( a ) Displacement spectrum of the two orthogonal fundamental modes of a nanowire ( R ≈100 nm, L ≈40 μm) for different powers of the feedback beam at vacuum condition (10 −4 Pa). ( b ) Simultaneous cooling of four distinguished resonances of the nanowire in vacuum with phase and gain optimized for more efficient cooling on one mode per pair. The displacement spectrum data in the absence of feedback is in red and the trace with feedback cooling is in blue. ( c ) Effective temperature of the first vibrational mode as a function of feedback laser power at ambient (red) and vacuum (blue) conditions. The solid line represents the theory assuming a linear relation between laser power and feedback gain g . ( d ) Effective temperature of the first (dark-green) and second (light-green) vibrational modes as a function of the phase of the feedback signal. Phases of −90° and 90° correspond to maximum oscillation amplification and maximum cooling, respectively. The solid lines represent the theory predictions. The error bars in c , d are estimated based on error propagation in the Lorentzian fit of the amplitude noise. Full size image SNR enhancement To measure the SNR in the transient regime, a 0.1-ms-long signal modulated at the mechanical frequency is sent to the nanowire right after the feedback is turned off (see Fig. 1a,c ). At the moment the signal arrives, with the feedback just switched off, the nanowire will also begin to thermalize at the rate of its mechanical dissipation, γ m . Provided the signal time ( τ sig ) is much shorter than the re-thermalization time , the measurement of the signal will not be significantly affected by thermal noise. Under vacuum conditions the mechanical dissipation rate of the nanowire is lower than 1 kHz, allowing integration times up to 1-ms long. We integrate the energy of the signal after introducing the impulsive force and compare it with the thermal noise to estimate the SNR in the presence and absence of periodic cooling. As we outlined earlier, linear feedback can also be simulated off-line using estimation techniques. We have performed both Kalman filtering and virtual feedback cooling (see Methods) on data taken in the absence of feedback. The digital Kalman filter is constructed based on prediction and update stages. At the prediction stage, the model of the system is used to estimate the evolution of the system for a short time into the future. In the update stage, the actual measurement results and known measurement and process noise vectors are used to refine the estimated evolution. The update stage of the filter is switched off when the impulsive force arrives, and the sizes of signal and noise are calculated as the phase-space distance between the measured and estimated trajectories in the presence and absence of the impulsive force. The virtual cooling method is used to directly simulate ideal periodic feedback cooling. A comparison of the estimation techniques with physical cooling in the transient regime is shown in Fig. 3a–c . Physical feedback cooling is shown to be as effective as the virtual cooling, which indicates nearly optimal actuation of the nanowire. For integration times longer than 0.4 ms, feedback cooling shows slightly higher improvement than virtual cooling. This is likely because of perturbation of the system parameters by laser noise within the timescale of mechanical decay time. The Kalman filter is shown to outperform both physical and virtual cooling. In all cases, the SNR degrades with a rate corresponding to the mechanical decay time as the thermal noise contribution increases. The SNR enhancement factor η SNR , defined as the ratio between the estimated SNR and that of the raw data where no cooling or filtering is used, is plotted in Fig. 3b . An enhancement factor of >5 has been observed for both the virtual cooling and Kalman filter methods. 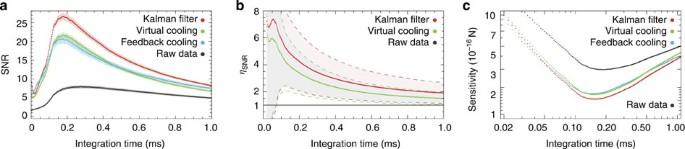Figure 3: Comparison of force measurement results of feedback cooling and estimation methods. (a) SNR measurement of energy of nanowire driven with impulsive photothermal force. The black and blue traces show the SNR measurement without and with feedback cooling. The red trace is the SNR of non-cooled data after post processing using the Kalman filter. The green trace represents the results of virtual cooling on data. The shaded regions represent the s.e. (b) The SNR enhancement factor,ηSNR, defined as the ratio of the estimated SNR divided by the SNR of the raw data. The dashed lines represent the s.d. in enhancement estimation. (c) Force resolution as a function of integration time for filtered, raw and feedback cooling data. Figure 3: Comparison of force measurement results of feedback cooling and estimation methods. ( a ) SNR measurement of energy of nanowire driven with impulsive photothermal force. The black and blue traces show the SNR measurement without and with feedback cooling. The red trace is the SNR of non-cooled data after post processing using the Kalman filter. The green trace represents the results of virtual cooling on data. The shaded regions represent the s.e. ( b ) The SNR enhancement factor, η SNR , defined as the ratio of the estimated SNR divided by the SNR of the raw data. The dashed lines represent the s.d. in enhancement estimation. ( c ) Force resolution as a function of integration time for filtered, raw and feedback cooling data. Full size image We note here that, while estimation methods can provide similar or even higher SNR enhancement factors than feedback cooling for short integration times, they require precise knowledge of system dynamics and parameters, and the production of the desired outcome can become computationally expensive. As an example we noticed that changing the mechanical frequency in the model by even 0.1% could significantly change the SNR. Such a change in frequency can occur easily through a change in the bulk temperature of the oscillator. To calculate the minimum force that can be measured with our set-up, we consider the response x ( t ) to a monochromatic force with magnitude F 0 , duration τ sig and frequency ω 0 /2 π that is , where χ ( t ) is the mechanical susceptibility. The mean squared displacement (for integration time τ ) is ; therefore, the force required to obtain a given mean squared displacement is This suggests a sensitivity as low as 2 × 10 −16 N after integration time of less than 0.1 ms for data filtered by the Kalman method. After 0.1 ms, the signal is switched off, so the relative contribution from the thermal noise increases and the sensitivity degrades. The high resolution and fast force sensing are important factors for biosensing where conformational changes typically happen on micro- to millisecond timescales [29] . In summary, we have demonstrated simultaneous active cooling of fundamental and higher-order modes of a bimetallic nanowire by means of optically induced thermal forces, obtaining temperatures as low as 8±1 K. In the transient regime, we investigated the effect of feedback cooling on the detection of an impulsive signal to demonstrate enhancement in measurement sensitivity. Although virtual feedback and estimation theories applied to off-line data provide similar improvements in sensitivity, they require the system parameters to be well known and constant, which may be a limitation in practical sensing applications. These technologies are increasingly important for sensing applications ranging from monitoring intermolecular interactions [29] to subsurface imaging [2] , and generally provide an alternative to passive cooling for systems that cannot be refrigerated. Both active feedback and numerical post-processing methods can be used to obtain an improvement in sensitivity over short time windows, especially advantageous when the system dynamics are changing rapidly and long integration times are not accessible [30] . Feedback cooling The power spectrum of the measured displacement of the nanowire driven by thermal forces in the presence of feedback is [12] where g is the effective gain that depends on the electronic gain, the mechanical quality factor, the thermal relaxation time and the induced mechanical rigidity resulting from photothermal forces [22] , ω m /2 π is the mechanical frequency, typically around 300 kHz, γ m /2 π is the mechanical linewidth, ranging from ~10 kHz in air down to 0.8 kHz in vacuum, m is the nanowire’s effective mass, ~1 pg, k B is the Boltzmann constant and T 0 is the initial temperature. The vibration of the nanowire introduces phase modulation on the reflected light. We send the DC homodyne signal to a piezo-actuated mirror to lock the phase of the local oscillator beam to that of the signal reflected from the nanowire. Above the locking bandwidth, which was ~10 kHz, the error signal then becomes a readout of the nanowire motion. The effective temperature and mechanical damping rates when feedback is sent to the nanowire are given by T eff = T 0 /(1+ g ) and γ eff =(1+ g ) γ m , respectively. The displacement spectrum has to be calibrated to compensate for the conversion and operational efficiency of the measurement devices. This is carried out by the integration of the area beneath the spectrum at room temperature and comparing it with the result expected from the equipartition theorem. For higher gains, a correction term [31] needs to be applied to the power spectrum (see Supplementary Note 4 ) and the effective temperature inferred. The latter is then characterized by a lower bound, , which depends on the spectral density of the detection noise S det . The lower the measurement noise and the mechanical linewidth are, the lower the minimum temperature achievable will be. Once this limit is reached, increasing the gain further results in noise squashing [31] , [32] (see Supplementary Note 4 and Supplementary Fig. 5 ). Data processing To measure the SNR, four sets of homodyne signals are recorded at a rate of 25 MS s −1 , in the presence and absence of feedback and in the presence and absence of the impulsive force. We then apply a spectral filter to restrict the signal to a 40-kHz bandwidth around the mechanical frequency. To calculate the SNR of, for example, feedback cooling data, we integrate the energy of the homodyne signal corresponding to the data taken in the presence of both periodic feedback and the impulsive force, and divide it by the average integral of the energy corresponding to data taken in the presence of periodic feedback and absence of the impulsive force. Analogous methods are used to measure SNR in the absence of feedback cooling, and when estimation techniques are used in place of physical cooling. All results are averaged over 150 traces, with the error calculated using s.e. (for Fig. 3a ) or s.d. (for Fig. 3b ). Estimation We use two different estimation strategies based on the discrete extended Kalman filter (EKF) [33] and the virtual cooling method [18] to enhance the SNR (refer to Supplementary Note 5 for more details). To identify the state-transition matrix of the EKF, we need to know the natural frequency, damping rate, initial amplitude, initial velocity, time interval, process and measurement noise vectors and initial covariance estimates. In order to propagate the state and estimate the evolution of the system, we use the Runge-Kutta (or RK4) method to predict the state of the system in the next step and update the system’s quadratures according to the relative uncertainties of measured and predicted values. We switch off the updating step of the EKF after 1 ms, at the time when the impulsive force arrives, so that the EKF predicts the subsequent behaviour of the system. This prediction is expected to be reliable while the system is not significantly affected by stochastic thermal noise, and deviations from it indicate the presence of the impulsive signal. The SNR is calculated in the same way as for feedback cooling, but instead of integrating the energy of the oscillator we integrate the phase-space distance between the observed and predicted trajectories. The virtual cooling is applied as suggested in the Supplementary Information of ref. 18 in order to simulate the periodic feedback cooling scheme. Knowing the mechanical susceptibility of the system we perform temporal discretization of the resulting Fredholm equation into a 1,000 × 1,000 matrix equation. Solving this yields the simulated measurement record, from which the SNR is calculated (refer to Supplementary Note 5 for more details). How to cite this article: Hosseini, M. et al. Multimode laser cooling and ultra-high sensitivity force sensing with nanowires. Nat. Commun. 5:4663 doi: 10.1038/ncomms5663 (2014).